Ultrafast charge and discharge biscrolled yarn supercapacitors for textiles and microdevices Flexible, wearable, implantable and easily reconfigurable supercapacitors delivering high energy and power densities are needed for electronic devices. Here we demonstrate weavable, sewable, knottable and braidable yarns that function as high performance electrodes of redox supercapacitors. A novel technology, gradient biscrolling, provides fast-ion-transport yarn in which hundreds of layers of conducting-polymer-infiltrated carbon nanotube sheet are scrolled into ~20 μm diameter yarn. Plying the biscrolled yarn with a metal wire current collector increases power generation capabilities. The volumetric capacitance is high (up to ~179 F cm −3 ) and the discharge current of the plied yarn supercapacitor linearly increases with voltage scan rate up to ~80 V s −1 and ~20 V s −1 for liquid and solid electrolytes, respectively. The exceptionally high energy and power densities for the complete supercapacitor, and high cycle life that little depends on winding or sewing (92%, 99% after 10,000 cycles, respectively) are important for the applications in electronic textiles. Supercapacitor electrodes having engineered hierarchical structures on nano- and micro-scales can provide high energy and power densities as a result of large surface-to-volume ratios, appropriately interconnected porosity and exploitation of both non-Faradaic and Faradaic charge storage processes [1] . Important recent advances in the micro-supercapacitor field have exploited novel active materials, such as carbon nanotubes (CNTs) [2] , reduced graphene oxide [3] , activated carbon [4] , conducting polymers [5] , [6] and metal oxides [7] . Many methods for fabricating miniature energy storage devices, such as rolling thin films into nanotubes [8] , [9] and micro-patterning [4] , [5] , [6] , [10] , [11] , [12] require micro-electromechanical system technology, which is expensive and difficult to upscale. Also, maintaining high energy and power densities under conditions where micro-supercapacitors are subjected to various bending and stretching deformations remains a challenge. Strong, flexible yarn-based supercapacitors are attractive as power sources for miniaturized electronic devices [13] , [14] , [15] , [16] such as micro-robots, wearable electronic textiles and implantable medical devices, as they can have small volumes and could be easily integrated into variously shaped structures. However, technical challenges have limited the development of strong, flexible and weavable yarns and fibres having attractive supercapacitor performance. Previously developed yarn supercapacitors have been based on solution-spun CNT/polymer fibres [17] and dry-spun CNT fibres [18] , which have lower energy storage capabilities than redox materials such as conducting polymers and metal oxides. Pseudocapacitors (redox supercapacitors) combine non-Faradic double-layer charge storage processes with redox reactions to achieve high effective capacitances and high energy storage densities [19] . However, while pseudocapacitors can provide higher energy storage capabilities than double-layer supercapacitors when drawn power is low, delivery of high energy at high power is a special problem unless the active material layer is very thin [20] , [21] . The use of very-thin active material depositions on much thicker current collectors can provide high energy and power densities based on active material volume or weight that are unrealistic predictors of the gravimetric or volumetric performance of the complete supercapacitor [22] . We here describe weavable, braidable, sewable and knottable yarn electrodes for redox supercapacitors that provide the combination of high energy storage densities and high rate capacities based on total cell volume. These yarns are made by a process called biscrolling, which involves inserting twist in a host sheet that is overlaid with guest. In previous work on making biscrolled yarns that are superconductors or electrodes for either batteries or fuel cells [23] , a CNT sheet host was overcoated with a layer of guest particles or nanofibres, and then twist spun to make a strong hybrid yarn that can contain 95 wt% of powder. These guest particles are trapped in scroll corridors of the nanotube host that are formed by inserting twist in the bilayer stack, but can remain highly electrochemically accessible because of yarn porosity and 100 micron or smaller yarn diameters. Preparation of two-ply yarn/metal wire assemblies In the present work, carbon multiwalled nanotube (MWNT) bundles in the host sheet are conformally overcoated with guest before twist insertion, which decreases the degree of segregation of the host and the guest into layers. Even though the guest interpenetrates the host nanotube sheet (or sheet stack), there is a gradient in guest concentration from sheet outer surface to sheet bottom ( Fig. 1a ). By using this modified biscrolling method (presently named gradient biscrolling), increased yarn strength resulted, as both host and guest structurally reinforce the yarn. The high mechanical strength and flexibility of the biscrolled yarns enable fabrication of weavable two-ply yarn/metal wire assemblies that exhibit high volumetric and areal energy and power densities in both liquid and solid electrolytes. While other configurations can also be usefully exploited, the present yarn supercapacitors use identical anodes and cathodes. 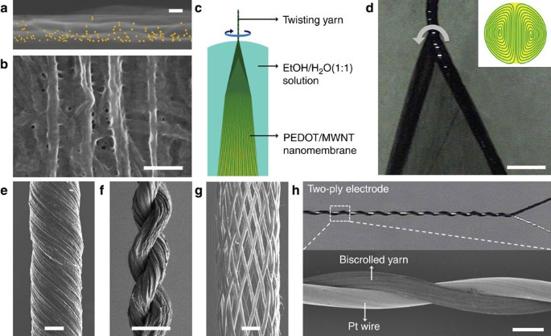Figure 1: The biscrolling method, precursors and derived structures for PEDOT/MWNT yarns. (a) An EDAX (energy-dispersive analysis by X-ray) map of the cross-section of a PEDOT-infiltrated two-layer CNT sheet stack, where PEDOT location is indicated by yellow dots signifying that sulphur concentration in above a threshold. Scale bar, 50 nm. (b) SEM image of the side of a PEDOT-coated MWNTs nanomembrane that was on top during PEDOT deposition. Scale bar, 200 nm. (c) Schematic illustration showing the fabrication of a biscrolled PEDOT/MWNT yarn. (d) Optical microscope image of the spinning wedge, which shows the wedge edges being twisted to form a dual-Archimedean scroll yarn, which is schematically illustrated in the inset. Scale bar, 200 μm. (e) SEM images of a biscrolled yarn with ~37° bias angle. Scale bar, 10 μm. (f) SEM image of two PEDOT/MWNT yarns plied together. Scale bar, 50 μm. (g) SEM image of a braided structure containing 32 biscrolled yarns. Scale bar, 100 μm. (h) Two SEM images of a PEDOT/MWNT biscrolled yarn that is plied with a 25 μm Pt wire. Scale bar, 40 μm. Figure 1: The biscrolling method, precursors and derived structures for PEDOT/MWNT yarns. ( a ) An EDAX (energy-dispersive analysis by X-ray) map of the cross-section of a PEDOT-infiltrated two-layer CNT sheet stack, where PEDOT location is indicated by yellow dots signifying that sulphur concentration in above a threshold. Scale bar, 50 nm. ( b ) SEM image of the side of a PEDOT-coated MWNTs nanomembrane that was on top during PEDOT deposition. Scale bar, 200 nm. ( c ) Schematic illustration showing the fabrication of a biscrolled PEDOT/MWNT yarn. ( d ) Optical microscope image of the spinning wedge, which shows the wedge edges being twisted to form a dual-Archimedean scroll yarn, which is schematically illustrated in the inset. Scale bar, 200 μm. ( e ) SEM images of a biscrolled yarn with ~37° bias angle. Scale bar, 10 μm. ( f ) SEM image of two PEDOT/MWNT yarns plied together. Scale bar, 50 μm. ( g ) SEM image of a braided structure containing 32 biscrolled yarns. Scale bar, 100 μm. ( h ) Two SEM images of a PEDOT/MWNT biscrolled yarn that is plied with a 25 μm Pt wire. Scale bar, 40 μm. Full size image More specifically, the biscrolled yarns were prepared by twist insertion in 100 nm thick conducting-polymer-infiltrated MWNT sheets ( Fig. 1a and Supplementary Fig. S1 ). The guest MWNT aerogel sheet strips were drawn from special CNT forests that are drawable [24] , and the conducting polymer yarn guest was subsequently deposited by vapour phase polymerization (VPP), which is a well-known method for providing uniform coatings of highly conducting polymer layers on substrates [25] . In the present case, the coated substrate structure is three-dimensional, as the conducting polymer coats MWNTs and MWNT bundles within the host sheet. The utilized conducting polymer, poly(3,4-ethylenedioxythiophene) (PEDOT), is well known to be useful as the active material for supercapacitor electrodes, as it is highly conducting, can charge both Faradaically and non-Faradaically, has high stability in the oxidized state [26] , and can be conveniently deposited. Scanning electron microscope (SEM) images indicate that the oriented fibular structure of the nanotube sheet is retained after VPP ( Fig. 1b ). The thickness of membranes comprising aligned PEDOT-coated MWNTs was controlled by varying the PEDOT loading level resulting from VPP; for 75 wt% PEDOT, the average nanomembrane thickness was ~102 nm ( Supplementary Fig. S2 ). PEDOT-coated nanotubes have been previously investigated as supercapacitor electrodes [27] , but complete supercapacitors were not demonstrated (so performance metrics based on total capacitor volume could not be obtained). Also, no work has been done using solid-state electrolytes, which are prerequisite for textile applications. The PEDOT/MWNT nanomembrane was biscrolled into yarn by using a novel method for twist insertion. This method provides one solution to the problem of exploiting wet-based processing of nanotube sheets into bilayers and then into biscrolled yarn without producing surface-tension-caused collapse of nanoscale thick membranes into highly irregular yarns before twist insertion. Two nanotube sheets are successively drawn from a nanotube forest and mechanically attached to a glass slide to provide a two-layer sheet stack. Without disturbing this attachment, the catalyst-containing solution was deposited on the sheet stack and dried, the PEDOT-conducting polymer was deposited by VPP and the film was washed in ethanol. Afterward, in a key step, an ethanol/water solution was used to float the hybrid nanomembrane from the substrate (except for a substrate-attached end that serves as an anchor, thereby enabling twist insertion in this membrane using a rotational electric motor ( Fig. 1c ). A wedge structure forms as the hybrid nanomembrane is twist spun into yarn ( Fig. 1d ). Opposite lateral sides of the wedge scroll in opposite directions to produce dual-Archimedean scrolls (the dark lines at spinning wedge edges in the Fig. 1c illustration and the Fig. 1d photograph). These interconnected scrolls, which are the three-dimensional analogue of a Cornu spiral ( Fig. 1d , inset), finally twist together to form an exotic type of two-ply yarn, which has only recently been discovered [23] . SEM images of the biscrolled yarn provided the yarn bias angle α , which is the angle between the yarn direction and the orientation direction of helically wrapped nanotubes on the outer yarn surface, which ranged in our experiments between ~22° and ~40°. For supercapacitor evaluations, biscrolled yarns with a bias angle of ~30° were usually used. About 8,000 turns per metre of inserted twist was needed to obtain this bias angle for a biscrolled 20 μm diameter yarn. Biscrolling generates high compressive forces [23] . As a result, compact PEDOT/MWNT multilayer structures having an important degree of porosity were formed within the biscrolled yarn ( Fig. 1e ). The surface porosity of the biscrolled yarn was found to decrease approximately proportionately with increase of PEDOT content ( Supplementary Fig. S3 ). The high mechanical strength (367±113 MPa), useful modulus (5.9±1.4 GPa) ( Supplementary Fig. S4 ) and flexibility of biscrolled yarns enabled fabrication of two-ply yarns and 32-yarn braids ( Fig. 1f ). Fast charge/discharge of two-ply electrodes in liquid and solid electrolytes A biscrolled PEDOT/MWNT yarn was plied with a Pt wire current collector to fabricate the identical electrodes used as both anode and cathode ( Fig. 1h ). Measurements of electrochemical performance were conducted using either a 1 M H 2 SO 4 liquid electrolyte or a solid poly(vinyl alcohol) (PVA–H 2 SO 4 ) electrolyte. Unless otherwise noted, the investigated biscrolled yarn has ~20 μm diameter and a two-ply electrode means a biscrolled yarn plied with an ~25 μm diameter Pt wire current collector. The solid-state supercapacitors were fabricated by separately infiltrating Pt-wire-plied PEDOT/MWNT yarn anode and cathode with ~10 μm average thickness of PVA–H 2 SO 4 . Two such electrodes were then plied together ( Supplementary Fig. S5 ) and then dried for 3 days at room temperature to provide fibre supercapacitors that are several centimeters in length. 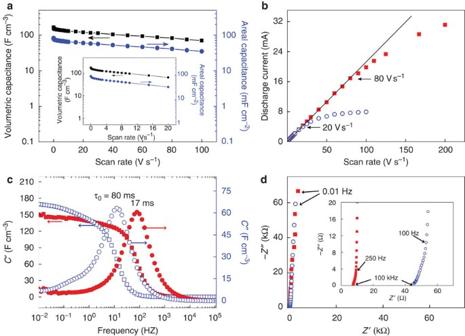Figure 2: Electrochemical performance of biscrolled yarn electrodes in solid and liquid electrolytes. (a) Volumetric and areal capacitances as a function of scan rate for two-ply yarn/wire supercapacitor electrodes (20 μm yarn diameter) in (a) liquid electrolyte, and inset, solid electrolyte, respectively. (b) Discharge current versus voltage scan rate for a two-ply supercapacitor electrode. The linear dependence of discharge current on scan rate up to high scan rates indicates ultra-high power ability in both liquid (filled red squares) and solid (open blue circles) electrolytes. (c) Frequency dependence of the real and imaginary parts (C′ andC′′) of the volumetric capacitance of a two-ply electrode supercapacitor using liquid (filled red circles) and solid (open blue circles) electrolytes. (d) Nyquist plots for two-ply yarn electrodes in liquid (filled red squares) and solid (open blue circles) electrolyte, showing the imaginary part versus the real part of impedance. Inset: magnified diagram for high frequencies. Figure 2a shows volumetric and areal capacitances as a function of scan rate from 0.01 V s −1 to 100 V s −1 for symmetric-electrode supercapacitors containing electrodes obtained by plying the Pt wire current collector and an ~20 μm biscrolled yarn. Here and elsewhere, unless otherwise noted, capacitances are single-electrode values that are normalized with respect to the area or volume of the electrochemically active material (presently the PEDOT/MWNT yarn). At a scan rate of 0.01 V s −1 , the volumetric capacitance of the liquid electrolyte (~167 F cm −3 ) is lower than that in the solid electrolyte (~180 F cm −3 ). However, the capacitance in the liquid electrolyte exceeded the capacitance in the solid electrolyte for scan rates above 1 V s −1 . Volumetric capacitances of ~147 F cm −3 (liquid electrolyte) and ~145 F cm −3 (solid electrolyte) were realized for a potential scan rate of l V s −1 , which decreased to ~129 F cm −3 and ~97 F cm −3 , respectively, when the scan rate was increased to 10 V s −1 . Using the total volume of both electrodes (including the Pt wire current collector) and the 10 V s −1 scan rate, the volumetric capacitances were 13 F cm −3 and 10 F cm −3 for liquid and solid electrolytes, respectively. These capacitances are at least six times higher than obtained at this scan rate for micro-supercapacitors using onion-like carbon electrodes [10] (1.1 F cm −3 ) or activated carbon [10] (1.5 F cm −3 ). Length-normalized capacitances for yarn supercapacitors, which are important for textile applications, were essentially the same at a 1 V s −1 scan rate for liquid (0.47 mF cm −1 ) and solid electrolytes (0.46 mF cm −1 ). Increasing scan rate to 10 V s −1 slightly decreased these capacitance (to 0.41 mF cm −1 and 0.31 mF cm −1 for the liquid and solid electrolytes, respectively). Absolute capacitance scaled linearly with supercapacitor length to a maximum capacitance of 10 mF for the longest device produced to date ( Supplementary Fig. S6 ). Figure 2: Electrochemical performance of biscrolled yarn electrodes in solid and liquid electrolytes. ( a ) Volumetric and areal capacitances as a function of scan rate for two-ply yarn/wire supercapacitor electrodes (20 μm yarn diameter) in ( a ) liquid electrolyte, and inset, solid electrolyte, respectively. ( b ) Discharge current versus voltage scan rate for a two-ply supercapacitor electrode. The linear dependence of discharge current on scan rate up to high scan rates indicates ultra-high power ability in both liquid (filled red squares) and solid (open blue circles) electrolytes. ( c ) Frequency dependence of the real and imaginary parts ( C ′ and C ′′) of the volumetric capacitance of a two-ply electrode supercapacitor using liquid (filled red circles) and solid (open blue circles) electrolytes. ( d ) Nyquist plots for two-ply yarn electrodes in liquid (filled red squares) and solid (open blue circles) electrolyte, showing the imaginary part versus the real part of impedance. Inset: magnified diagram for high frequencies. Full size image The performance of the biscrolled yarn supercapacitor was also higher than for conducting polymer and carbon-ink-based solid-electrolyte supercapacitors [6] , [15] , [28] . As recent high-performance supercapacitors are made of nanometre-thick active materials on much larger volume substrates, normalization based on electrode geometrical area is here used to provide fair performance comparisons. Meng and Ding [28] reported that polypyrrole-decorated nanoporous gold membrane supercapacitors with a thickness of ~100 nm (HClO 4 /PVA gel electrolyte) had an areal capacitance of 1.8 mF cm −2 at 0.1 V s −1 . Wang et al . [6] showed that polyaniline nanowire micro-supercapacitors with a thickness of ~400 nm (H 2 SO 4 /PVA gel electrolyte) had a capacitance of 23.5 mF cm −2 at 0.1 mA cm −2 . Also Fu et al . [15] reported areal capacitance (9.5 mF cm −2 ) for a fibre supercapacitor with ~21 μm thickness of ink-deposited carbon (H 2 SO 4 /PVA gel electrolyte) on a 150 μm diameter nickel wire, which was packaged using a plastic tube for a flexible/wearable energy device. The two-ply electrode supercapacitor presented here has a capacitance of 73 mF cm −2 at 1 V s −1 that is at least three times higher than for the previously described supercapacitors. Although the PEDOT undergoes changes in volume changes and electrical conductivity during redox reaction [29] , cyclic voltammograms were rectangular in shape even at low scan rates, indicating capacitive behaviour ( Supplementary Fig. S6a ). Little reduction in capacitance was observed even for scan rates as high as ~25 V s −1 and ~5 V s −1 in liquid and solid electrolytes, respectively ( Supplementary Fig. S7a,b ). This low dependence of capacitance on scan rate is similar to that for conventional double-layer supercapacitors having much lower volumetric capacitances. Discharge current for the two-ply electrodes was a linear function of potential scan rate at up to ~80 and ~20 V s −1 in liquid and solid electrolyte, respectively ( Fig. 2b ). The discharge rate capability of the two-ply electrode supercapacitor can also be evaluated from the relaxation time constant ( τ 0 ), which is ~17 ms for the two-ply electrode supercapacitor in the aqueous electrolyte ( Fig. 2c ). This time constant is smaller than that for the onion-like carbon (26 ms) and activated carbon (700 ms) supercapacitors [10] . The time constant for solid-electrolyte supercapacitors ( Fig. 2c ) was significantly longer (~80 ms), which can be explained by an increased equivalent series resistance (ESR). This increased ESR is mostly due to an increased equivalent distributed resistance, which relates to the diffusion of ions within the porous electrode [30] ( Fig. 2d ). High cyclic life and stability of two-ply electrodes in a solid electrolyte Biscrolled yarn supercapacitors (comprising two-ply anode and cathode separated by solid electrolyte) were stable in ambient atmosphere and showed high cycle life even when bent, helically wound or woven into a glove. The results in Fig. 3a show that the desired rectangular dependence of current density on applied potential was retained for scan rates up to 1 V s −1 . The results in Fig. 3b–d show little change in capacitance when the capacitor was bent (~2% for 2,000 cycles), helically wound on a glass capillary tube (~8% for 10,000 cycles) or woven into a glove (~1% for 10,000 cycles), respectively. Bending did increase the ESR compared with that for the unbent state, which may limit charge/discharge rates ( Supplementary Fig. S8b ). 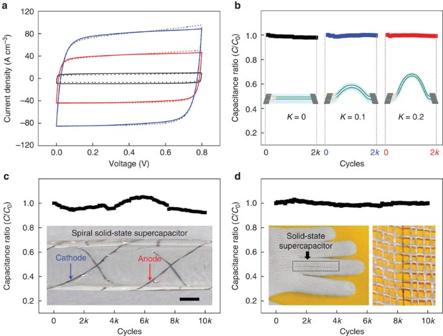Figure 3: Cyclic life and stability of solid-electrolyte biscrolled yarn supercapacitors. (a) Cyclic voltammetry at different voltage scan rates of 0.1 V s−1(black line), 0.5 V s−1(red line) and 1 V s−1(blue line) for the solid-electrolyte, biscrolled yarn supercapacitor in ambient atmosphere (solid line). Exposure of the supercapacitor in ambient atmosphere for 3 months (dotted line) did not significantly change in performance. Normalized capacitance in ambient atmosphere (C/Co, whereCois the initial capacitance) versus cycle number for a two-ply, all-solid-state Pt/yarn supercapacitor after deformation by (b) bending on a flexible polyethylene terephthalate film (κis curvature in mm−1); (c) winding on a 1.4 mm diameter glass tube. Scale bar, 500 μm. (the inset shows a photograph taken after solid-electrolyte coating); and (d) weaving into a glove (the yarn supercapacitor was 5 cm long). Figure 3: Cyclic life and stability of solid-electrolyte biscrolled yarn supercapacitors. ( a ) Cyclic voltammetry at different voltage scan rates of 0.1 V s −1 (black line), 0.5 V s −1 (red line) and 1 V s −1 (blue line) for the solid-electrolyte, biscrolled yarn supercapacitor in ambient atmosphere (solid line). Exposure of the supercapacitor in ambient atmosphere for 3 months (dotted line) did not significantly change in performance. Normalized capacitance in ambient atmosphere ( C / C o , where C o is the initial capacitance) versus cycle number for a two-ply, all-solid-state Pt/yarn supercapacitor after deformation by ( b ) bending on a flexible polyethylene terephthalate film ( κ is curvature in mm −1 ); ( c ) winding on a 1.4 mm diameter glass tube. Scale bar, 500 μm. (the inset shows a photograph taken after solid-electrolyte coating); and ( d ) weaving into a glove (the yarn supercapacitor was 5 cm long). Full size image Energy and average power densities for the complete system for commercialization For a given constant scan rate v (V s −1 ), the average power during discharge ( P av , in W) was calculated by integrating the current density ( I ) versus voltage ( V ) curves: where V i is the initial voltage during discharge. Integration to obtain average power during charge and discharge provided nearly identical results. The discharged energy ( E , in Wh) was obtained using equation (3): The combination of exceptional energy storage and power densities for the complete supercapacitor (including both electrodes of plied yarn/Pt wire and solid electrolyte) is indicated in the Ragone plots of Fig. 4 , which compares performance with that for other micro-size energy storage devices. The yarn supercapacitor (using 20 μm diameter biscrolled yarn) had an average power density of 40 W cm −3 , which is about four times higher than for commercial 25 mF supercapacitors [10] . The biscrolled yarn supercapacitor exhibited energy densities of up to 1.4 mWh cm −3 , which is over two times higher than for commercial micro-supercapacitors [10] , [31] . Although a commercial 500 μAh lithium thin-film battery [10] delivers much high energy, it has three orders of magnitude lower power density than for the biscrolled yarn redox supercapacitor. Also the biscrolled yarn redox supercapacitor has two orders of magnitude higher power density and a six times higher energy density than for a recent all-solid-state, flexible supercapacitor based on MnO 2 -coated carbon fibre. [32] These total cell volume comparisons avoid the pitfall [22] of studies that report high active-material energy and power densities by using small amounts of active material on comparatively massive current collectors. By plying the active yarn with current collecting wire and using the nanotubes to provide enhanced electronic connectivity down to the nanoscale, we decrease electrode weight and volume by eliminating the need for a conventional conducting binder, which can also interfere with electrochemical accessibility. Multifunctionality is deployed: the solid electrolyte functions as separator and connector, the scrolled nanotubes provide electrical, electrochemical and mechanical functions, and the PEDOT provides both energy storage and mechanical reinforcement. 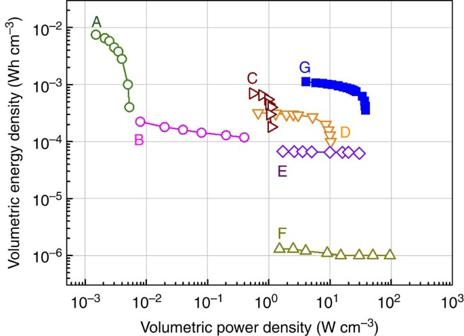Figure 4: Volumetric energy and average power densities for complete supercapacitors. Ragone plots comparing volumetric energy and average power densities for the present all-solid-state, two-ply electrode supercapacitor (G) (yarn diameter, 20 μm) with that for a commercially available 4 V/500 μAh Li thin-film battery10(A), a 2.75 V/44 mF activated carbon electrochemical capacitor31(C), a 3.5 V/25 mF supercapacitor10(D), a 63 V/220 μF electrolytic capacitor10(E), a 3 V/300 μF Al electrolytic capacitor31(F), as well as an experimental MnO2carbon fibre supercapacitor32(B). Figure 4: Volumetric energy and average power densities for complete supercapacitors. Ragone plots comparing volumetric energy and average power densities for the present all-solid-state, two-ply electrode supercapacitor (G) (yarn diameter, 20 μm) with that for a commercially available 4 V/500 μAh Li thin-film battery [10] (A), a 2.75 V/44 mF activated carbon electrochemical capacitor [31] (C), a 3.5 V/25 mF supercapacitor [10] (D), a 63 V/220 μF electrolytic capacitor [10] (E), a 3 V/300 μF Al electrolytic capacitor [31] (F), as well as an experimental MnO 2 carbon fibre supercapacitor [32] (B). Full size image Such attractive electrochemical performance is attributed to the good adhesion and resulting low contact resistance between the biscrolled yarn and the Pt wire current collector, as well as the topology of the biscrolled yarn. The strong physical contact caused by compressive forces generated during plying results in a low ESR [33] . The ESR measured dramatically decreased from 110.4 to 8.5 Ω (at 1 kHz) when an unplied biscrolled electrode was replaced by an electrode of yarn plied with Pt wire, and this resistance decrease can also be seen in the decrease of the diameter of the Nyquist semi-circle ( Supplementary Fig. S8a ). The latter can be related to the decrease of charge transfer resistance between the yarn and the Pt wire. We also demonstrated the effect of yarn geometry on supercapacitor performance. 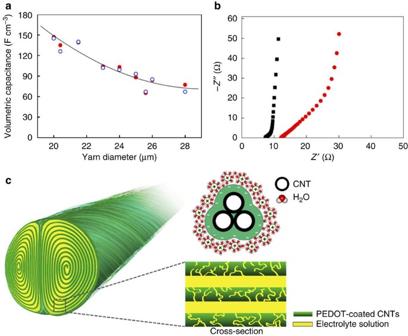Figure 5: Yarn diameter effects and structure for PEDOT/MWNT yarn supercapacitors. (a) The dependence of volumetric capacitance (for a scan rate of 1 V s−1) on yarn diameter for a two-ply electrode supercapacitor in solid (open blue circles) and liquid (filled red circles) electrolytes. (b) Nyquist plots for two-ply yarn/wire electrodes using different diameter PEDOT/MWNT yarn. The ESR measured at 1 kHz for a 20 μm diameter yarn (filled black squares) is 8.5 Ω, which is ~2 times smaller than that of a 28 μm diameter yarn (filled red circles) at this frequency (16.2 Ω). (c) Schematic illustration of the pore structure of MWNT/PEDOT biscrolled yarns and the electrochemical double layer of a PEDOT-coated MWNT bundle. Figure 5a shows the dependence of volumetric capacitance on yarn diameter for two-ply yarn electrodes measured at 1 V s −1 scan rate are nearly identical for liquid and solid electrolytes, and both monotonically increased by a factor of about 2 upon decreasing yarn diameter from 28 to 20 μm. The yarn diameter was controlled by the hybrid nanomembrane width and the forest height. Otherwise, the hybrid membranes were identically prepared with the same amount of inserted twist per yarn length and all yarns contained about 75 wt% PEDOT. The origin of this strong diameter dependence of volumetric capacitance is not completely understood. A number of effects might be important, increasing yarn diameter (while applying the same twist per yarn length) can cause yarn densification that closes pore space between biscrolled sheets and from one biscrolled layer to another, which when filled with electrolyte provide valuable ion-transport pathways from yarn surface to yarn centre. Increased yarn diameter would also increase ion diffusion distances [23] , even if yarn pore structure is unaffected. Additionally, Hertzian contact pressure theory for cylindrical yarns held in parallel or in contact with metal wires of constant diameter, predicts lower contact pressure for large diameter yarns for the same contact force conditions [34] . Decreased contact pressure can generate increased contact resistance, thereby resulting in an increase of the ESR. In fact, the ESR measured at 1 kHz decreased from 16.2 to 8.5 Ω for two-ply electrode supercapacitors when the diameter of the yarn decreased from 28 to 20 μm ( Fig. 5b ). Evaluation of longer lengths of plied yarn electrodes showed only small reduction in capacitance ( Supplementary Fig. S9 ), suggesting the potential for scale up, although batch fabrication processes currently limit obtainable lengths. Figure 5: Yarn diameter effects and structure for PEDOT/MWNT yarn supercapacitors. ( a ) The dependence of volumetric capacitance (for a scan rate of 1 V s −1 ) on yarn diameter for a two-ply electrode supercapacitor in solid (open blue circles) and liquid (filled red circles) electrolytes. ( b ) Nyquist plots for two-ply yarn/wire electrodes using different diameter PEDOT/MWNT yarn. The ESR measured at 1 kHz for a 20 μm diameter yarn (filled black squares) is 8.5 Ω, which is ~2 times smaller than that of a 28 μm diameter yarn (filled red circles) at this frequency (16.2 Ω). ( c ) Schematic illustration of the pore structure of MWNT/PEDOT biscrolled yarns and the electrochemical double layer of a PEDOT-coated MWNT bundle. Full size image The explanation for the extraordinary combination of high power and high energy storage capabilities lies in the novel structure of the biscrolled yarn ( Fig. 5c ). Even though there is up to 75 wt% PEDOT in the biscrolled yarn, the scroll structure provides a continuous pathway for both ion and electronic transport from yarn surface to yarn centre, as well as sufficient porosity through scroll layers for cross-layer ion transport. The ease of ion transport is enhanced by the gradient in PEDOT concentration through the thickness of the nanomembrane that is twist spun to make the biscrolled yarn. As a result, one side of each of the hundreds of scroll layers in a 20 μm diameter biscrolled yarn is largely free of PEDOT, and therefore able to provide fast ion transport via incorporated electrolyte. In conclusion, this method for producing biscrolled yarn electrodes seems amenable to upscaling. As drawable nanotube forest could be continuously grown on a flexible belt (like a flexible steel foil coated with oxide and catalyst) [35] and drawn at high rates into sheet, continuous transfer of nanotubes from forest on one belt to sheet on a second moving belt seems feasible. After liquid-based deposition of catalyst on the nanotube sheet and VPP deposition of the PEDOT on the second moving belt, a delivered liquid could be used to separate the bilayer sheet from the belt substrate for conventional twist insertion to make yarn. The described technology of gradient biscrolling has produced supercapacitor yarns whose hierarchal structure leads to outstanding energy storage and power performance as a redox supercapacitor. These weavable, sewable, braidable and knottable yarns are promising for electronic textile applications, as the fabrication process seems upscalable and supercapacitor performance is little affected by bending or weaving. The high strength of the biscrolled yarns means that textiles woven from these yarns could simultaneously provide structural reinforcement and energy storage, such as in automotive panels. On the opposite extreme, it was demonstrated that all-solid-state supercapacitors can be sewn as a single thread into textiles to power micro-electronic devices. Materials Drawable MWNT forests (~400 μm high and consisting of ~12 nm diameter nanotubes that contain ~9 walls and form large bundles) were grown on a Si wafer by chemical vapour deposition, as previously described [23] . PVA ( M w 146,000–186,000), iron(III) p -toluenesulfonate hexahydrate (Fe(III)PTS), pyridine (anhydrous, 99.8% purity), 1-butanol (≥99% purity) and 3,4-ethylenedioxythiophene (EDOT, 97% purity) were from Sigma-Aldrich Corporation and 1 M aqueous sulphuric acid solution was from Daejung Chemicals and Metals Company. SEM and AFM images of the PEDOT-infiltrated MWNT sheets are shown in Supplementary Figs S1 and S2 . PEDOT/MWNT nanomembrane preparation A 20 wt% solution of iron (III) p -toluenesulfonate hexahydrate (Fe(III)PTS) in butanol (with 1.6 volume % of subsequently added pyridine) was used as oxidizing agent for the polymerization of PEDOT (after diluting this stock solution to obtain 4–16 wt% of oxidant). The diluted solutions were added drop-wise over a two-layer stack of aligned CNT aerogel sheet strips that were supported by a glass substrate, and then the sheet stack was dried at 60 °C for 20 min. Densification during evaporation of the solution reduced the stack thickness to ~75 nm. VPP to provide PEDOT infiltration within the nanotube host sheets was accomplished by exposing these catalyst-containing sheets to EDOT vapour in a VPP chamber for 1 h at 60 °C. After the VPP, the PEDOT-coated nanotube sheets were washed three times with ethanol. Fabrication of yarn electrodes Biscrolled yarn was fabricated from a PEDOT-infiltrated nanotube sheet strip using the process illustrated in Fig. 1c . The hybrid nanomembrane sheet strips were released from a supporting glass substrate by using a 50/50 by volume ethanol/water solution. While one end of the 7.5 cm long sheet strip remained attached to the substrate, the opposite strip end was peeled from the substrate and attached on an electric motor shaft with a flat rectangular paddle. Then, the nanomembrane was slowly twisted using the motor to introduce ~8,000 turns per metre of inserted twist per yarn length ( Supplementary Movie 1 ). After twist insertion, both ends of the biscrolled yarn were fixed to the glass slide using carbon tape and the biscrolled yarn was dried at room temperature. Depending upon the thickness and width of the hybrid nanomembrane, the resulting yarn diameter ranged from ~20 to ~35 μm. Two-ply electrodes for supercapacitors were made by twisting together a PEDOT/MWNT biscrolled yarn and an ~25 μm Pt wire using an electric motor ( Supplementary Movie 2 ). The electrodes contained 5.7 μg of active materials (PEDOT and MWNT) per cm length. Preparation of solid electrolyte Water (30 ml) and sulphuric acid (1.67 ml) were mixed using a stirring bar for 10 min in a 50 ml glass bottle (1 M sulphuric acid solution). Three grams of PVA ( M w 146,000–186,000) was added in the solution, and then the mixture was stirred for 1 h at ~90 °C. This solution was deposited and dried, as described above, to obtain the solid electrolyte. Calculation of yarn porosity The fraction of void space in the yarn that is potentially available for electrolyte filling was calculated by using the following equation: where V v is the void-space volume, V t is the total volume of the yarn, V m = V p + V c ) is the volume of materials in the yarn, including PEDOT and MWNT. The MWNT volume ( V c ) was calculated by dividing MWNT mass by the density of MWNT bundles (~1.67 g cm −3 ). The PEDOT volume ( V p ) was calculated by dividing the PEDOT mass by PEDOT density, using 1.47 g cm −3 for the density of PEDOT [36] . Sheet stack mass was measured before and after PEDOT coating using a microbalance to obtain the wt% of PEDOT in the yarn. Calculated porosities are given in Supplementary Fig. S3 . Apparatus for characterizations Surface morphology and height profiles of hybrid nanomembranes were characterized using scanning electron microscopy (Hitachi S4700) and atomic force microscopy (Park Systems XE-100). Cyclic voltammetry and electrochemical impedance spectroscopy (EIS) measurements were obtained using electrochemical analysers (CHI 627B from CH Instruments and Reference 600 from Gamry Instruments). Mechanical properties of the yarn micro supercapacitor ( Supplementary Fig. S4 ) were characterized using a Thermal Mechanical Analyzer (TMA/SS7100 from RT Instruments). Construction of supercapacitors Supercapacitors were constructed using two configurations. For tests in liquid electrolytes, two identically prepared electrodes were immersed in a beaker of the electrolyte. The electrodes were constructed from biscrolled yarn plied with thin platinum wire. For solid-state devices, two such electrodes were first individually coated with 1 M H 2 SO 4 /PVA gel electrolyte to avoid short circuit in the next step ( Supplementary Fig. S5a ). After a few hours of drying in air, the full two-electrode system was made by plying together the individual electrodes prepared in the previous step. After immersion of the two-electrode yarn in the gel electrolyte and thoroughly drying the electrolyte in air, the solid-state supercapacitor could be directly woven into a textile structure without the need of further packaging ( Supplementary Fig. S5b ). Calculation of the electrochemical capacitance for two-ply electrode supercapacitors Electrochemical characterizations of the supercapacitor yarns are given in Supplementary Figs S6–S9 . Cyclic voltammetry curves were obtained at the scan rate from 0.01 V s −1 to 100 V s −1 . EIS was conducted for frequencies between 100 kHz and 10 mHz using a 5 mV AC voltage and a 0.1 V DC voltage. EIS tests were made in 1 M sulphuric acid electrolyte using a symmetric two-electrode system. Except for the results in Supplementary Fig. S7 , the capacitance for the two-electrode system ( C ) was derived using the time-integrated current and the voltage scan range from cyclic voltammogram curves. For Supplementary Fig. S7 , C = I /(d V /d t ), where I is the discharge current. Using these values of C , the single-electrode volumetric capacitance ( C sp ) was calculated from the following equation [37] : where V vol is the total volume of the electrochemically active material in both electrodes. The factor of 4 multiplier adjusts the capacitance of the two-electrode system and the combined volume of two electrodes to the capacitance and volume of a single electrode. Calculation of the real and imaginary parts of electrochemical capacitance for two-ply electrode supercapacitors The frequency dependence of the real and imaginary parts ( C′ and C ′′) of electrochemical capacitance was obtained from electrochemical impedance spectroscopy measurements by using the following equations [38] : where ω is the angular frequency and Z′ and Z′′ are the real and imaginary parts of the impedance, defined as Z′ ( ω ) 2 + Z′′ ( ω ) 2 =| Z ( ω )| 2 . How to cite this article: Lee, J.A. et al . Ultrafast charge and discharge biscrolled yarn supercapacitors for textiles and microdevices. Nat. Commun. 4:1970 doi: 10.1038/ncomms2970 (2013).